Light-regulated gene repositioning inArabidopsis Plant genomes are extremely sensitive to, and can be developmentally reprogrammed by environmental light cues. Here using rolling-circle amplification of gene-specific circularizable oligonucleotides coupled with fluorescence in situ hybridization, we demonstrate that light triggers a rapid repositioning of the Arabidopsis light-inducible chlorophyll a / b -binding proteins ( CAB) locus from the nuclear interior to the nuclear periphery during its transcriptional activation. CAB repositioning is mediated by the red/far-red photoreceptors phytochromes (PHYs) and is inhibited by repressors of PHY signalling, including COP1, DET1 and PIFs. CAB repositioning appears to be a separate regulatory step occurring before its full transcriptional activation. Moreover, the light-inducible loci RBCS , PC and GUN5 undergo similar repositioning behaviour during their transcriptional activation. Our study supports a light-dependent gene regulatory mechanism in which PHYs activate light-inducible loci by relocating them to the nuclear periphery; it also provides evidence for the biological importance of gene positioning in the plant kingdom. Changes in light quality and quantity trigger rapid alterations in gene expression and consequently lead to dramatic modifications in plant morphology and physiology [1] . For example, during seedling development, initial exposure to light turns on the photoautotrophic developmental programme called photomorphogenesis via massive transcriptional reprogramming [2] , [3] , [4] . A major class of light-induced nuclear genes encodes essential components of the chloroplast photosynthetic machinery, such as the chlorophyll a / b -binding proteins (CABs) [4] . Although a suite of photoreceptors and their signalling components have been identified for mediating light responses, the mechanism by which light orchestrates complex developmental programmes such as photomorphogenesis is still poorly understood [3] . Accumulating evidence from studies in yeast and metazoan models suggests that the organization of the genome, and in particular the spatial positioning of individual genes to distinct subnuclear compartments, plays an important role in cellular programming [5] , [6] , [7] . As the divergence of the plant kingdom predates the divergence of the fungal and metazoan lineages [8] , the general principles of gene positioning in yeast and metazoan models might not be conserved in plants. Therefore, we asked whether light regulates developmental programming by reorganizing the spatial positioning of individual light-responsive genes. Compared with yeast and metazoan models, little is known about the positioning of individual genes in plants. A key obstacle for gene positioning studies in plants has been difficulty in labelling a single endogenous gene locus [9] . Although fluorescence in situ hybridization (FISH) has been successfully used in plants to study the organization of repetitive DNA and chromatin regions spanning more than 100 kb (refs 10 , 11 , 12 , 13 ), conventional FISH does not efficiently label DNA regions of 10 kb or less; therefore, it does not have the resolution to detect positional changes of single genes. In addition to FISH, the Lac operator/Lac repressor reporter system [14] has also been used to visualize chromatin dynamics in transgenic plant lines [15] , [16] , [17] . However, because inserting a reporter construct into a specific locus in Arabidopsis remains challenging [18] , and because tandem repeat sequences tend to cluster together and thus could potentially alter the endogenous chromosomal organization at the transgene locus in Arabidopsis [19] , this reporter system has not been particularly useful to study the chromatin dynamics of specific endogenous loci. Here we present a new protocol to label individual endogenous gene loci in Arabidopsis nuclei by using rolling-circle amplification of gene-specific padlock probes coupled with FISH. Using this new approach, we demonstrate that light triggers a rapid repositioning of the light-inducible CAB locus from the nuclear interior to the nuclear periphery during its transcriptional activation. CAB repositioning is regulated by the red (R)/far-red (FR) photoreceptors phytochromes (PHYs) and PHY-signalling components. In addition, CAB repositioning appears to be a separate regulatory step occurring before its full transcriptional activation. Moreover, the light-inducible loci RBCS ( Rubisco small subunit ), PC ( Plastocyanin ) and GUN5 ( Genomes uncoupled 5 ) undergo similar repositioning behaviour on their activation. Our data support a light-dependent gene regulatory mechanism in which PHYs activate light-inducible loci by relocating them to the nuclear periphery. Labelling of individual genes using padlock FISH We developed a protocol to label individual gene loci in plant nuclei based on an in situ genotyping method for human cells established by Nilsson and coworkers [20] . This method uses rolling-circle amplification of gene-specific circularizable oligonucleotides—‘padlock’ probes—coupled with FISH ( Fig. 1a and see Methods ). To demonstrate that the padlock FISH protocol works for Arabidopsis nuclei, we first tested whether we could use the protocol to detect the centromeric 180-bp repeats [21] . We designed a padlock probe recognizing the 30-bp centromere sequence immediately flanking the HindIII site ( Fig. 1a and Supplementary Table S1 ). Then, we tested whether the 180-bp repeat signals from padlock FISH were co-localized with immunolocalization signals for the centromeres, which were labelled using anti-HTR12 antibodies against CENH3 (ref. 22 ). As shown in Fig. 1b , 92.9% of the 180-bp FISH signals ( n =435) were at least partially overlapping with a CENH3 signal, suggesting that the padlock FISH protocol can effectively label the 180-bp repeats. To show that the protocol also works for a single-gene locus, we chose the UBQ11 (At4g05050) locus. Because UBQ11 lies within the pericentromeric region on chromosome 4 (ref. 23 ), we expected that the UBQ11 locus should also be associated with a centromere. Indeed, the UBQ11 padlock FISH signals were always closely associated with a CENH3 signal ( Fig. 1c ); the average distance from the UBQ11 signal to the closest CENH3 signal was 0.37±0.13 μm ( n =30, mean±s.d.). Together, these results demonstrate that in principle, the padlock FISH protocol can be used to determine the position of both repetitive sequences and single-gene loci in plant nuclei. 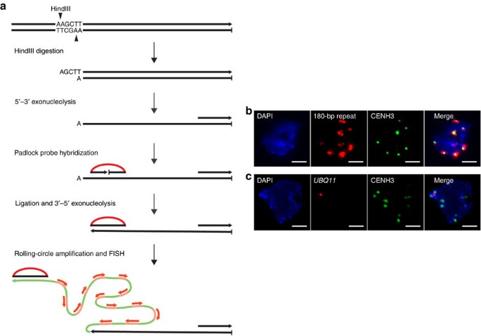Figure 1: Labelling of centromeric 180-bp satellite repeats and theUBQ11locus using padlock FISH. (a) Schematic illustration of the padlock FISH protocol using the 180-bp repeat probe as a model. The illustration is modified from figure 1 of Larssonet al.20First, the target DNA is digested by HindIII (see the list of enzymes used for other padlock probes used in this study inSupplementary Table S1) and subsequently by lambda 5′–3′ exonuclease to generate single-stranded DNA flanking the HindIII site. The padlock probes, which contain target sequences near the HindIII site and a ‘detection probe’ sequence (shown in red, seeSupplementary Table S1), are annealed to the target DNA and the ends of the probes are joined by ligation. Then, phi29 DNA polymerase is added. The 3′–5′ exonuclease activity of the polymerase removes the 3′-protruding sequence beyond the padlock probe, and then the polymerase uses the circularized probe as the template and amplifies its DNA by rolling-circle amplification. The amplified DNA product is detected by hybridization of fluorescent-labelled oligonucleotides (shown in red, see ‘detection probes’ inSupplementary Table S1). Arrowheads indicate the 3′ ends, and bars indicate the 5′ ends. (b) Representative images showing the localization of centromeric 180-bp repeats (red) labelled by padlock FISH and centromeres (green) by immunolocalization using anti-HTR12 antibodies against CENH3 in nuclei from cotyledons of 4-day-old Col-0 seedlings grown in R light. The nuclei were counterstained with DAPI (blue). (c) Representative images showing the localization of theUBQ11locus (red) labelled by padlock FISH and centromeres (green) by immunolocalization using anti-HTR12 antibodies in nuclei from cotyledons of 4-day-old Col-0 seedlings grown in R light. The nuclei were counterstained with DAPI (blue). Scale bars, 2 μm. Figure 1: Labelling of centromeric 180-bp satellite repeats and the UBQ11 locus using padlock FISH. ( a ) Schematic illustration of the padlock FISH protocol using the 180-bp repeat probe as a model. The illustration is modified from figure 1 of Larsson et al . [20] First, the target DNA is digested by HindIII (see the list of enzymes used for other padlock probes used in this study in Supplementary Table S1 ) and subsequently by lambda 5′–3′ exonuclease to generate single-stranded DNA flanking the HindIII site. The padlock probes, which contain target sequences near the HindIII site and a ‘detection probe’ sequence (shown in red, see Supplementary Table S1 ), are annealed to the target DNA and the ends of the probes are joined by ligation. Then, phi29 DNA polymerase is added. The 3′–5′ exonuclease activity of the polymerase removes the 3′-protruding sequence beyond the padlock probe, and then the polymerase uses the circularized probe as the template and amplifies its DNA by rolling-circle amplification. The amplified DNA product is detected by hybridization of fluorescent-labelled oligonucleotides (shown in red, see ‘detection probes’ in Supplementary Table S1 ). Arrowheads indicate the 3′ ends, and bars indicate the 5′ ends. ( b ) Representative images showing the localization of centromeric 180-bp repeats (red) labelled by padlock FISH and centromeres (green) by immunolocalization using anti-HTR12 antibodies against CENH3 in nuclei from cotyledons of 4-day-old Col-0 seedlings grown in R light. The nuclei were counterstained with DAPI (blue). ( c ) Representative images showing the localization of the UBQ11 locus (red) labelled by padlock FISH and centromeres (green) by immunolocalization using anti-HTR12 antibodies in nuclei from cotyledons of 4-day-old Col-0 seedlings grown in R light. The nuclei were counterstained with DAPI (blue). Scale bars, 2 μm. Full size image Light-dependent repositioning of the CAB locus To test whether light regulates the spatial organization of individual genes, we turned to some of the best-characterized light-induced genes, the CAB genes. Three members of the CAB gene family, CAB1-3 (At1g29930, At1g29920 and At1g29910), are clustered in a 7-kb region on chromosome 1, hereafter referred to as the CAB locus ( Supplementary Fig. S1 ). In mesophyll cells, all three CAB genes are repressed in the dark and are rapidly induced by light via the R and FR photoreceptors PHYs [24] , [25] . To study CAB positioning specifically in the mesophyll nuclei, we first characterized the nuclear morphology of various cell types and defined the criteria to identify mesophyll cell nuclei among isolated nuclei ( Supplementary Fig. S2 and Supplementary Discussion ). We then asked whether the CAB locus is found at distinct subnuclear positions between the inactive state in the dark (D) and the active state in the light. Using a padlock probe specific to the CAB1-3 genes ( Supplementary Fig. S1 and Supplementary Table S1 ), we found a dramatic difference in the radial distribution of the CAB locus in mesophyll nuclei between D and monochromatic R or FR light conditions ( Fig. 2a ). In the dark, when the CAB genes are repressed, the CAB locus was localized in the nuclear interior ( Fig. 2a ). In striking contrast, in R or FR light, when the genes were activated, the distribution of CAB loci peaked near the nuclear periphery; this phenomenon was more pronounced in R light than in FR light ( Fig. 2a ). We arbitrarily defined the area within 0.2 μm of the nuclear edge as the ‘nuclear peripheral zone’ and calculated the percentage of CAB loci localized to the nuclear peripheral zone with s.e. from two or three biological replicates in each condition. The percentage of CAB loci localized to the nuclear peripheral zone increased drastically from 21±3% ( n =140) in D to 35±3% ( n =124) in FR light and 49±4% ( n =153) in R light ( Fig. 2a ). This increase in the percentage of CAB loci at the nuclear periphery correlates with an increase in the expression of CAB in FR and R compared with D ( Fig. 2b ). In contrast, the distribution of a light-independent control gene locus, PP2A (protein phosphatase 2A, At1g69960), was not altered by light ( Supplementary Fig. S3 ). Together, these results indicate that the CAB locus is repositioned from the nuclear interior to the nuclear periphery during transcriptional activation by R and FR light. 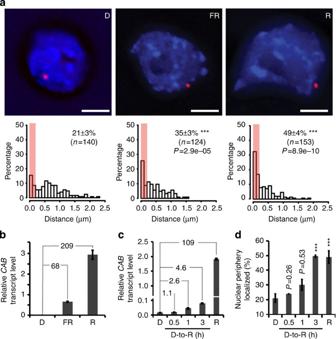Figure 2: Repositioning of theCABlocus from the nuclear interior to the nuclear periphery during light activation. (a) Representative images ofCABpositioning (top) and distribution of theCABlocus (bottom) relative to the nuclear edge in mesophyll cell nuclei from 4-day-old Col-0 seedlings grown in the dark (D), far-red (FR), and red (R) light. TheCABlocus was labelled using padlock FISH (red) and the nuclei were counterstained with DAPI (blue). Scale bars, 2 μm (in the images). The pink areas in theCABdistribution panels represent the nuclear peripheral zone—the region 0.2 μm or closer to the nuclear edge—and the average percentage ofCABloci within the nuclear peripheral zone with s.e. from three independent replicates is shown in each panel. ‘n’ represents the total number of padlock FISH signals analysed from all replicates. TheCABdistribution data from the R and FR samples were compared with that of the D sample using Welch’s two-samplet-test, ***P<0.001. (b) qRT–PCR analysis ofCAB1-3messenger RNA levels from seedlings grown in D, FR or R light. Transcript levels were calculated relative to those ofPP2A. Fold-changes ofCABexpression in R or FR relative to D conditions are shown. Error bars represent s.d. from three replicates. (c) Relative expression levels ofCABsduring the D-to-R transition. Fold-changes ofCABexpression in R-treated samples relative to that in the dark are shown. Error bars represent s.d. from three replicates. (d) Average percentage ofCABloci at the nuclear periphery at the indicated time points during the D-to-R transition. Error bars in paneldrepresent s.e. calculated from three independent replicates (except for the 0.5-h time point, which had two replicates). TheCABdistribution data from the D-to-R transition samples were compared with that of the D sample using Welch’s two-samplet-test, ***P<0.001. Figure 2: Repositioning of the CAB locus from the nuclear interior to the nuclear periphery during light activation. ( a ) Representative images of CAB positioning (top) and distribution of the CAB locus (bottom) relative to the nuclear edge in mesophyll cell nuclei from 4-day-old Col-0 seedlings grown in the dark (D), far-red (FR), and red (R) light. The CAB locus was labelled using padlock FISH (red) and the nuclei were counterstained with DAPI (blue). Scale bars, 2 μm (in the images). The pink areas in the CAB distribution panels represent the nuclear peripheral zone—the region 0.2 μm or closer to the nuclear edge—and the average percentage of CAB loci within the nuclear peripheral zone with s.e. from three independent replicates is shown in each panel. ‘ n ’ represents the total number of padlock FISH signals analysed from all replicates. The CAB distribution data from the R and FR samples were compared with that of the D sample using Welch’s two-sample t -test, *** P <0.001. ( b ) qRT–PCR analysis of CAB1-3 messenger RNA levels from seedlings grown in D, FR or R light. Transcript levels were calculated relative to those of PP2A . Fold-changes of CAB expression in R or FR relative to D conditions are shown. Error bars represent s.d. from three replicates. ( c ) Relative expression levels of CABs during the D-to-R transition. Fold-changes of CAB expression in R-treated samples relative to that in the dark are shown. Error bars represent s.d. from three replicates. ( d ) Average percentage of CAB loci at the nuclear periphery at the indicated time points during the D-to-R transition. Error bars in panel d represent s.e. calculated from three independent replicates (except for the 0.5-h time point, which had two replicates). The CAB distribution data from the D-to-R transition samples were compared with that of the D sample using Welch’s two-sample t -test, *** P <0.001. Full size image We then measured the kinetics of CAB repositioning when dark-grown seedlings were first exposed to light ( Fig. 2c,d ). The percentage of CAB loci at the nuclear periphery was rapidly increased from 21±3% in D to 49±1% ( n =170 mean±s.e. of three independent replicates, two-sample t -test, P <0.001) within 3 h of R light exposure ( Fig. 2d ). These data further show that on light induction, the CAB locus is rapidly relocated from the nuclear interior to the nuclear periphery. Again, the expression level of the CAB genes correlated closely with the percentage of CAB loci at the nuclear periphery ( Fig. 2c,d ), further supporting the notion that the repositioning of the CAB locus to the nuclear periphery is associated with its transcriptional activation. Interestingly, although it took only 3 h for the percentage of peripherally localized CAB loci to reach the same level as that in continuous R light ( Fig. 2d ), the expression level of the CAB genes was still far below the fully activated level in continuous R light ( Fig. 2c ). These data suggest that CAB repositioning is a separate regulatory step that occurs before its full transcriptional activation. CAB repositioning is triggered by PHYs It has been shown that the activation of CAB expression is dependent on the R and FR photoreceptors, the PHYs. In Arabidopsis , PHYA and PHYB are the prominent photoreceptors in sensing continuous monochromatic FR and R light, respectively; CAB activation is almost completely abolished in the phyA-211 mutant in continuous FR light and in the phyB-9 mutant in continuous R light ( Fig. 3a,b ) [25] , [26] . To test whether CAB repositioning is also PHY dependent, we examined CAB positioning in the phyA-211 and phyB-9 mutants. In agreement with the expression data, the CAB -repositioning response was also substantially diminished in phyA-211 in FR and in phyB-9 in R light ( Fig. 3c,d ), indicating that the light-dependent CAB repositioning response is mainly dependent on PHYA in continuous FR light and on PHYB in continuous R light. Consistent with this notion, YHBox, a line expressing a constitutively active PHYB mutant [27] , was able to activate CAB expression and trigger the repositioning of the CAB locus to the nuclear periphery in the dark ( Fig. 3e,f ). On the basis of these results, we conclude that light-dependent CAB repositioning to the nuclear periphery is mediated by the photoactivation of PHYs. 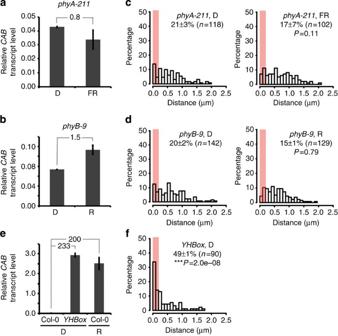Figure 3:CABrepositioning during light activation is PHY dependent. (a) qRT–PCR data showing theCAB1,2,3mRNA levels in 4-day-oldphyA-211seedlings grown in the D or FR light conditions. Transcript levels were calculated relative to those ofPP2A. Fold-change ofCABexpression in FR relative to D is shown. Error bars represent s.d. from three replicates. (b) qRT–PCR data showing theCAB1,2,3mRNA levels in 4-day-oldphyB-9seedlings grown in D or R light conditions. Transcript levels were calculated relative to those ofPP2A. Fold-change ofCABexpression in R relative to D is shown. Error bars represent s.d. from three replicates. (c) The distribution ofCABloci and the average percentages ofCABloci localized to the nuclear peripheral zone inphyA-211in either the D or FR light conditions. (d) The distribution ofCABloci and the average percentages ofCABloci localized to the nuclear peripheral zone inphyB-9in either the D or R light conditions. (e) qRT–PCR data showing theCAB1,2,3mRNA levels in 4-day-old Col-0 andYHBoxseedlings grown in the D and Col-0 seedlings in R light. Transcript levels were calculated relative to those ofPP2A. Fold-change ofCABexpression in D-grownYHBoxor R-grown Col-0 relative to that of D-grown Col-0 is shown. Error bars represent s.d. from three replicates. (f) The distribution ofCABloci and the average percentages ofCABloci localized to the nuclear peripheral zone inYHBoxseedlings grown in the D. TheCABdistribution data inc,dandfwere from two independent replicates, and ‘n’ represents the total number of padlock FISH signals analysed from all replicates. Statistical analyses between FR and D samples ofphyA-211, between R and D samples ofphyB-9and between D-grownYHBoxand Col-0 were performed using Welch’s two-samplet-test, and ***P<0.001. Figure 3: CAB repositioning during light activation is PHY dependent. ( a ) qRT–PCR data showing the CAB [1] , [2] , [3] mRNA levels in 4-day-old phyA-211 seedlings grown in the D or FR light conditions. Transcript levels were calculated relative to those of PP2A . Fold-change of CAB expression in FR relative to D is shown. Error bars represent s.d. from three replicates. ( b ) qRT–PCR data showing the CAB [1] , [2] , [3] mRNA levels in 4-day-old phyB-9 seedlings grown in D or R light conditions. Transcript levels were calculated relative to those of PP2A . Fold-change of CAB expression in R relative to D is shown. Error bars represent s.d. from three replicates. ( c ) The distribution of CAB loci and the average percentages of CAB loci localized to the nuclear peripheral zone in phyA-211 in either the D or FR light conditions. ( d ) The distribution of CAB loci and the average percentages of CAB loci localized to the nuclear peripheral zone in phyB-9 in either the D or R light conditions. ( e ) qRT–PCR data showing the CAB [1] , [2] , [3] mRNA levels in 4-day-old Col-0 and YHBox seedlings grown in the D and Col-0 seedlings in R light. Transcript levels were calculated relative to those of PP2A . Fold-change of CAB expression in D-grown YHBox or R-grown Col-0 relative to that of D-grown Col-0 is shown. Error bars represent s.d. from three replicates. ( f ) The distribution of CAB loci and the average percentages of CAB loci localized to the nuclear peripheral zone in YHBox seedlings grown in the D. The CAB distribution data in c , d and f were from two independent replicates, and ‘ n ’ represents the total number of padlock FISH signals analysed from all replicates. Statistical analyses between FR and D samples of phyA-211 , between R and D samples of phyB-9 and between D-grown YHBox and Col-0 were performed using Welch’s two-sample t -test, and *** P <0.001. Full size image CAB positioning is regulated by COP1, DET1 and PIFs To further confirm the role of PHY signalling in CAB positioning, we asked whether CAB positioning is regulated by known PHY-signalling components. PHY signalling has been extensively investigated, and many signalling components mediating the induction of CAB expression have been identified [3] , [4] . Among the positive factors involved in CAB expression is the master bZIP transcriptional regulator HY5 (elongated HYpocotyl 5), which is not essential for CAB induction but binds directly to a G-box in the promoter of the CAB genes and plays a role in the full activation of CAB expression in the light ( Fig. 4a ) [28] , [29] , [30] , [31] . Interestingly, in R light, CAB positioning in the hy5 mutant was statistically similar to that of Col-0 ( Fig. 4b ), indicating that HY5 does not play a major role in CAB repositioning. These data also imply that CAB repositioning and full activation could be regulated by distinct trans -factors. 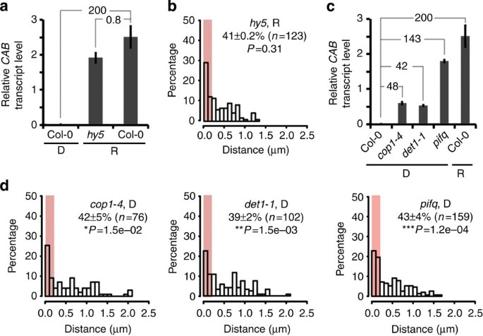Figure 4: TheCABrepositioning response in photomorphogenetic mutants. DET1, COP1 and PIFs, but not HY5, are involved in the regulation ofCABpositioning inArabidopsis. (a) Relative expression level ofCABsin Col-0 andhy5in R light and Col-0 in the D. Fold-changes ofCABexpression between R-grown and D-grown Col-0 and between R-grownhy5and Col-0 are shown. (b) Distribution ofCABloci and the average percentages of nuclear peripheral localizedCABloci in thehy5mutant grown in R light. Data were from two independent replicates, and ‘n’ represents the total number of padlock FISH signals analysed from both replicates. Statistical analyses using Welch’s two-samplet-test showed no significant difference between theCABdistributions inhy5and Col-0 in R light (P=0.31). (c) The relative expression level ofCABsincop1-4, det1-1 and pifqin D. Fold-changes ofCABexpression between the respective mutant and Col-0 are shown. (d) Distribution ofCABloci and the average percentage ofCABloci at the nuclear periphery in D-growncop1-4, det1-1andpifq.TheCABdistribution data were from at least two independent replicates, and ‘n’ represents the total number of padlock FISH signals analysed from independent replicates. Statistical analyses betweenCABdistribution data from each mutant and corresponding Col-0 control samples were performed using Welch’s two-samplet-test; *P<0.05, **P<0.01 and ***P<0.001. Error bars in panelsaandcrepresent s.d. from three replicates. Figure 4: The CAB repositioning response in photomorphogenetic mutants. DET1, COP1 and PIFs, but not HY5, are involved in the regulation of CAB positioning in Arabidopsis . ( a ) Relative expression level of CABs in Col-0 and hy5 in R light and Col-0 in the D. Fold-changes of CAB expression between R-grown and D-grown Col-0 and between R-grown hy5 and Col-0 are shown. ( b ) Distribution of CAB loci and the average percentages of nuclear peripheral localized CAB loci in the hy5 mutant grown in R light. Data were from two independent replicates, and ‘ n ’ represents the total number of padlock FISH signals analysed from both replicates. Statistical analyses using Welch’s two-sample t -test showed no significant difference between the CAB distributions in hy5 and Col-0 in R light ( P =0.31). ( c ) The relative expression level of CABs in cop1-4, det1-1 and pifq in D. Fold-changes of CAB expression between the respective mutant and Col-0 are shown. ( d ) Distribution of CAB loci and the average percentage of CAB loci at the nuclear periphery in D-grown cop1-4, det1-1 and pifq. The CAB distribution data were from at least two independent replicates, and ‘ n ’ represents the total number of padlock FISH signals analysed from independent replicates. Statistical analyses between CAB distribution data from each mutant and corresponding Col-0 control samples were performed using Welch’s two-sample t -test; * P <0.05, ** P <0.01 and *** P <0.001. Error bars in panels a and c represent s.d. from three replicates. Full size image A number of master repressors of PHY signalling have also been described, including DET1 (De-ETiolated 1) [32] , COP1 (COnstitutively Photomorphogenic) [33] and phytochrome interacting factors (PIFs) [34] . PIFs are master bHLH transcription factors that antagonize PHY-mediated light responses [34] ; COP1 and DET1 are substrate recognition subunits of CULLIN4 E3 ubiquitin ligase complexes [35] , [36] , which determine the abundance of key transcription factors including HY5 and the PIFs [37] , [38] . DET1 has also been implicated in chromatin modification [39] . Knocking out DET1 , COP1 or 4 PIF family members leads to constitutive photomorphogenetic responses in the dark, including the derepression of the CAB genes ( Fig. 4c ) [2] , [32] , [33] . We therefore examined CAB positioning in dark-grown det1-1 , cop1-4 and pifq mutants and asked whether the light-independent CAB activation in these mutants is accompanied by CAB localization to the nuclear periphery. As shown in Fig. 4d , the distribution of the CAB locus in det1-1 , cop1-4 and pifq in the dark was significantly different from that of dark-grown Col-0 and instead resembled that of Col-0 in R light. These results indicate that COP1, DET1 and the PIFs are essential for retaining the CAB locus in the nuclear interior in the dark. Interestingly, although cop1-4 and det1-1 showed similar CAB -positioning patterns as pifq , CAB expression levels in cop1-4 and det1-1 were considerably lower than that in pifq ( Fig. 4c,d ). These data are consistent with previous reports that COP1 and DET1, but not the PIFs, also play a positive role in the full activation of CAB expression in the light [28] , [33] . Our results provide a possible explanation for this phenomenon: COP1 and DET1 play opposing roles in repressing CAB repositioning and promoting full CAB activation, whereas PIFs are involved only in the repression of CAB positioning to the nuclear periphery. Together, these results further support the conclusion that CAB positioning is regulated by PHY signalling and begin to elucidate distinct roles of PHY signalling components in CAB positioning. Light-dependent repositioning of other light-inducible loci To test whether repositioning to the nuclear periphery is a common phenomenon among light-induced genes, we examined three additional light-induced photosynthesis-related genes, RBCS1A (At1g67090), GUN5 (At5g13630) and PC (At1g76100) ( Fig. 5a–c ), which are distributed throughout the Arabidopsis genome. As shown in Fig. 5d–f , all three loci were localized to the nuclear interior in the dark and to the nuclear periphery in the light, when they are transcriptionally activated. These results support the notion that relocating genes from the nuclear interior to the nuclear periphery is a common mechanism of gene activation by light. 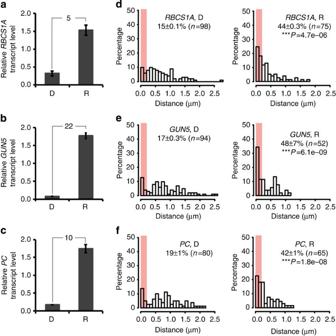Figure 5: Light-dependent repositioning of other light-inducible loci. (a) qRT–PCR results showing the relative expression levels ofRBCS1Ain 4-day-old Col-0 seedlings grown either in the D or R light conditions. Transcript levels were calculated relative to those ofPP2A. (b) qRT–PCR results showing the relative expression levels ofGUN5in 4-day-old Col-0 seedlings grown either in the D or R light conditions. Transcript levels were calculated relative to those ofPP2A. (c) qRT–PCR results showing the relative expression levels ofPCin 4-day-old Col-0 seedlings grown either in the D or R light conditions. Transcript levels were calculated relative to those ofPP2A. Error bars in panelsa,bandcrepresent s.d. from three replicates. (d) The distribution and the average percentage of peripherally localizedRBCS1Aloci in D and R conditions. (e) The distribution and the average percentage of peripherally localizedGUN5loci in D and R conditions. (f) The distribution and the average percentage of peripherally localizedPCloci in D and R conditions. The gene distribution data ind,eandfwere from two independent replicates, and ‘n’ represents the total number of padlock FISH signals analysed from all replicates. Statistical analyses between R and D samples for each gene were performed using Welch’s two-samplet-test, ***P<0.001. Figure 5: Light-dependent repositioning of other light-inducible loci. ( a ) qRT–PCR results showing the relative expression levels of RBCS1A in 4-day-old Col-0 seedlings grown either in the D or R light conditions. Transcript levels were calculated relative to those of PP2A . ( b ) qRT–PCR results showing the relative expression levels of GUN5 in 4-day-old Col-0 seedlings grown either in the D or R light conditions. Transcript levels were calculated relative to those of PP2A . ( c ) qRT–PCR results showing the relative expression levels of PC in 4-day-old Col-0 seedlings grown either in the D or R light conditions. Transcript levels were calculated relative to those of PP2A . Error bars in panels a , b and c represent s.d. from three replicates. ( d ) The distribution and the average percentage of peripherally localized RBCS1A loci in D and R conditions. ( e ) The distribution and the average percentage of peripherally localized GUN5 loci in D and R conditions. ( f ) The distribution and the average percentage of peripherally localized PC loci in D and R conditions. The gene distribution data in d , e and f were from two independent replicates, and ‘ n ’ represents the total number of padlock FISH signals analysed from all replicates. Statistical analyses between R and D samples for each gene were performed using Welch’s two-sample t -test, *** P <0.001. Full size image We have demonstrated that light triggers the repositioning of a group of light-inducible genes from the nuclear interior to the nuclear periphery during their transcriptional activation. Our experimental evidence supports a model in which PHY signalling regulates two separate regulatory steps during CAB induction: its repositioning and its full activation ( Fig. 6 ). This conclusion is supported by three lines of evidence: CAB repositioning to the nuclear periphery occurs before its full activation; the percentage of CAB loci at the nuclear periphery correlates closely with CAB ’s expression level; and CAB repositioning and its full transcriptional activation are regulated by distinct trans -factors. Although it is still not clear whether CAB repositioning is required for its full activation, our data suggest that the repositioning of individual genes to the nuclear periphery is an important regulatory step in light-regulated gene induction ( Fig. 6 ). 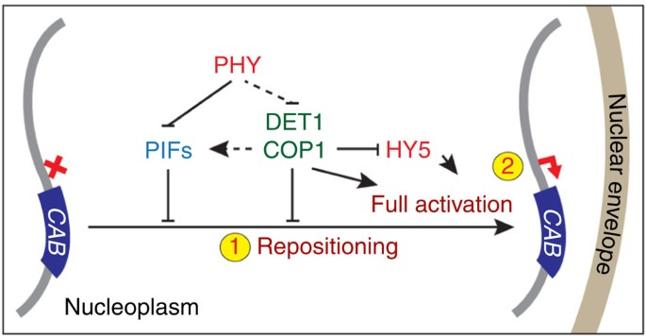Figure 6: Model forCABrepositioning and gene activation during its induction by light. The transcriptionally silencedCABlocus is localized to the nuclear interior. Light activates PHY signalling to trigger theCABlocus’ repositioning to the nuclear periphery and its full transcriptional activation. Although it is still not clear whetherCABlocalization to the nuclear periphery directly causes its activation,CAB’s repositioning and full activation appear to be separate steps.CABlocalization to the nuclear periphery is inhibited by COP1, DET1 and PIFs, whose functions are repressed by PHYs in the light. COP1 could inhibitCABrepositioning by stabilizing at least one of the PIFs, PIF3. Both DET1 and COP1 play separate and positive roles in the full activation step, which also requires HY5. Figure 6: Model for CAB repositioning and gene activation during its induction by light. The transcriptionally silenced CAB locus is localized to the nuclear interior. Light activates PHY signalling to trigger the CAB locus’ repositioning to the nuclear periphery and its full transcriptional activation. Although it is still not clear whether CAB localization to the nuclear periphery directly causes its activation, CAB ’s repositioning and full activation appear to be separate steps. CAB localization to the nuclear periphery is inhibited by COP1, DET1 and PIFs, whose functions are repressed by PHYs in the light. COP1 could inhibit CAB repositioning by stabilizing at least one of the PIFs, PIF3. Both DET1 and COP1 play separate and positive roles in the full activation step, which also requires HY5. Full size image Our study also provides key initial evidence supporting the biological significance of gene positioning in transcriptional regulation in the plant kingdom. The gene repositioning phenomenon of the light-induced genes examined here resembles the behaviour of a number of inducible genes in yeast, including INO1 , GAL1 , GAL2 , HSP104 and SUC2 , which relocate from the nucleoplasm to the nuclear periphery on activation [40] , [41] , [42] , [43] . Therefore, our results suggest that the basic principles of spatial organization of genes during transcriptional regulation might be part of an ancient regulatory mechanism that evolved before the divergence of the fungal/animal and plant lineages ~1.6 billon years ago [8] . Our findings that PHY-signalling components play distinct roles in CAB repositioning provide insight into the signalling pathways as well as the molecular mechanisms that regulate gene positioning in plants. Although many studies from yeast and metazoan models have shown the implications of gene repositioning in transcription, the molecular mechanisms of gene repositioning are still largely unknown. Studies of the INO1 gene in yeast have provided the most in-depth mechanism so far: gene positioning could be controlled by both cis -regulatory elements and trans -factors [44] , [45] , [46] . Our results suggest that the PIFs are potential trans -factors that retain light-inducible loci in the nuclear interior in the dark ( Fig. 6 ). A possible mechanism is that PIFs induce gene-silencing histone modifications at the target loci. Consistent with this hypothesis, a recent study showed that PIF3 directly binds to the G-box elements of light-inducible photosynthetic genes, including GUN5 and the CAB paralogue LHCB2.1 , and it promotes gene silencing by recruiting the histone deacetylase HDA15 (ref. 47 ). Further supporting this model, histone deacetylase 6, along with PHYB, is involved in light-dependent chromatin compaction in Arabidopsis [48] . DET1 could be another trans -factor that retains light-inducible genes in the nucleoplasm. Tomato DET1 binds to the nonacetylated amino-terminal tail of histone H2B [39] ; in addition, DET1 has been shown to act as a key transcriptional repressor [49] . Therefore, DET1 could work in concert with PIFs to retain light-inducible genes in the nuclear interior. CAB repositioning by light is probably triggered by the PHY-dependent degradation of PIFs [34] . Although the mechanism of PIF degradation is still largely unknown, COP1 has been shown to be required for PIF3 accumulation in the dark [38] . Therefore, both PHYs and COP1 might regulate gene positioning by controlling PIF abundance ( Fig. 6 ). Previous studies in yeast and metazoan systems also indicate that the nuclear pore complex plays an important role in promoting gene activation [35] , [36] , [37] . It remains to be investigated whether light-induced gene loci are directly associated with the nuclear pore complex in plants. All of the photosynthesis-regulated genes analysed here belong to a group of light-regulated genes that are induced during the dark-to-light transition and remain induced in the light. Although all four of these genes showed similar light-dependent repositioning behaviour, it is still far from sufficient to conclude that all light-induced genes relocate to the nuclear periphery in the light. It would not be surprising if different mechanisms are involved in the activation of different classes of light-inducible genes [2] . It would be interesting to examine the group of early light-induced genes [2] that are transiently induced by light during the dark-to-light transition and see whether these genes are only temporarily localized to the nuclear periphery during their activation. It also remains to be investigated whether light-repressed genes [2] are activated at the nuclear periphery in the dark. In addition, it is still not clear whether repositioning to the nuclear periphery is also involved in gene activation in other signalling pathways in plants. On the basis of the principles learned from yeast and metazoan models, there are different gene activating and silencing domains in the nucleus [5] , [6] , [7] ; therefore, we anticipate that more functional domains will also be defined in plant nuclei. A recent elegant study on the localization of FLC alleles suggests that gene repositioning is also involved in gene silencing in Arabidopsis [17] . We expect that our study on light-regulated gene repositioning and the padlock FISH method described here will stimulate further studies on genome organization in plants. Plant materials and growth conditions Wild-type Col-0, phyA-211 (ref. 50 ), phyB-9 (ref. 51 ), hy5 (ref. 52 ), cop1-4 (ref. 33 ), det1-1 (ref. 32 ) and pifq (ref. 53 ) were used to characterize CAB positioning. The YHBox line is a transgenic line carrying a 35S:YHB-YFP-FLAG construct in the phyB-9 mutant background; this line resembles the previously described constitutively active phyB allele, YHB [54] , but in the Col-0 background ( Supplementary Fig. S4 ). Arabidopsis seed sterilization, stratification and growth conditions were described previously [55] . Padlock FISH Plant fixation and isolation of nuclei were performed based on Schubert et al . [56] , and the padlock FISH procedure was developed based on Larsson et al . [20] with modifications. Seedlings grown for 100 h under the indicated conditions were fixed in cold fixation buffer (4% formaldehyde, 10 mM Tris–HCl pH 7.5, 10 mM EDTA, 100 mM NaCl) for 30 min under vacuum. Approximately 100 cotyledons were chopped in 50 μl lysis buffer (15 mM Tris–HCl pH 7.5, 2 mM EDTA, 0.5 mM spermine-4HCl, 80 mM KCl, 20 mM NaCl and 0.1% Triton X-100) with a razor blade on a slide. The resulting suspension containing the released nuclei was transferred into four volumes of nuclei suspension buffer (100 mM Tris–HCl pH 7.5, 50 mM KCl, 2 mM MgCl 2 , 5% sucrose and 0.05% Tween-20). The nuclear suspension was spotted on a slide and air-dried overnight at room temperature. The slides were either used immediately or stored at −20 °C. All subsequent steps were performed in a 55-μl SecureSeal chamber (Grace Bio-Labs, Bend, OR) and are illustrated in Fig. 1a . The nuclei were washed in PBS and permeabilized with PBS containing 0.2% Triton X-100. After two washes in PBS, the slides were incubated with a DNA digestion solution containing 0.5 U μl −1 of restriction enzyme (New England Biolabs, Ipswich, MA) at 37 °C for 30 min; the specific restriction enzymes used for each target gene are listed in Supplementary Table S1 . After two washes in buffer A (100 mM Tris–HCl pH 7.5, 150 mM NaCl and 0.05% Tween-20), the slides were treated with 0.2 U μl −1 of 5′–3′ Lambda exonuclease (New England Biolabs) in Lambda exonuclease buffer containing 0.2 μg μl −1 BSA and 10% glycerol at 37 °C for 30 min to generate a single-stranded target sequence ( Fig. 1a ). Then, the slides were briefly washed twice in buffer A and incubated with T4 ligase buffer supplemented with 0.1 μM gene-specific padlock probes ( Supplementary Table S1 ), 0.1 U μl −1 T4 ligase (New England Biolabs), 1 mM ATP, 250 mM NaCl and 0.2 μg μl −1 BSA. The ligation reaction was carried out at 37 °C for 30 min, which allowed the padlock probes to anneal to the target sequence and to circularize ( Fig. 1a ). After one wash in buffer B (2 × saline-sodium citrate buffer and 0.05% Tween-20), the slides were incubated in 1 U μl −1 of phi29 DNA polymerase (Fermentas, Burlington, Canada) in 1 × phi29 buffer supplemented with 0.25 mM dNTPs, 0.2 μg μl −1 BSA and 10% glycerol at 37 °C for 2 h. In this step, the padlock probe sequence was amplified by rolling-circle amplification ( Fig. 1a ). The slides were then incubated with 0.25 μM fluorescently tagged detection oligonucleotide probes ( Supplementary Table S1 ) in 2 × saline-sodium citrate buffer containing 20% formamide at 37 °C for 20 min. Unbound fluorescent probes were washed away with five washes in PBS with 0.05% Tween at 37 °C and three washes with PBS at room temperature. The nuclei were counterstained with 4′,6-diamidino-2-phenylindole (DAPI; 500 ng ml −1 ) at room temperature for 20 min, washed three times with water, mounted in Prolong Gold antifade reagent (Life Technologies, Carlsbad, CA) and sealed with fast-dry nail polish. On the basis of our experiments on the CAB and PP2A loci, and assuming that all nuclei were diploid, the detection efficiency for each experiment ranged from 4 to 7% of all potential target sequences. This detection efficiency is slightly lower than the 10% detection efficiency reported for animal cells [20] . Given that some of the nuclei could be polyploid, the actual detection efficiency of this method is expected to be a slightly lower than this range. As a result, there was only one padlock FISH signal in the majority of nuclei examined. Immunolocalization Antibodies used were rabbit polyclonal antisera against HTR12 (1:100), recognizing Arabidopsis CENH3 (ref. 22 ), and mouse monoclonal antibodies against the nuclear pore complex (1:250, QE5, recognizing Nup214, Nup153 and p62 of the mammalian nuclear pore complex, Covance, Princeton, NJ) [57] . Immunolocalization was performed as described previously [58] , [59] . For combined padlock FISH and immunolabeling, after the padlock FISH procedure, the slides were washed three times with PBS and blocked with PBS containing 3% BSA for 30 min at 37 °C. The slides were then incubated with primary antisera overnight at room temperature or at 37 °C. After five washes in PBS, the slides were incubated with secondary antibodies—either donkey-anti-mouse-AlexaFluor 488 or donkey-anti-rabbit-AlexaFluor 488 (Life Technologies, 1:300 dilution)—at 37 °C. The slides were washed five times in PBS and counterstained with 500 ng ml −1 DAPI. Fluorescence microscopy Mesophyll nuclei were selected based on their morphology as described in Supplementary Fig. S2 . Three-dimensional image stacks with a z -step size of 0.2 μm were acquired with a DeltaVision microscope system (Applied Precision, Issaquah, WA) consisting of an IX-71 Olympus inverted microscope (Olympus, Tokyo, Japan) with a UPLSAPO oil immersion objective lens (× 100, numerical aperture 1.40; Olympus) and a Coolsnap HQ2 high-resolution charge-coupled device camera. DAPI, AlexaFluor 488, CY3 and CY5 were detected with appropriate filters. The image stacks were deconvolved with a constrained iterative of 15 by using softWoRx software (Applied Precision) on an Octane Workstation (SGI, Mountain View, CA). Gene positioning measurements and data analysis To measure the distance from the padlock FISH signal of a gene locus to the nuclear edge, an optical section with the strongest and most focused padlock FISH signal was used. The nuclear edge was determined by DAPI intensity as described in Supplementary Fig. S5a,b and outlined using the two-dimensional polygon finder function in softWoRx ( Supplementary Fig. S5c,d ). Then, using the centre of the padlock FISH signal as the centre, a circle was drawn whose circumference intersected the nuclear edge ( Supplementary Fig. S5c ). The distance between the intersection point and the center of the padlock FISH signal was defined as the distance between the gene locus and the nuclear edge. For each light condition or genotype, at least two biological replicates were analysed. The data from all replicates were combined and the radial distribution of each gene locus was plotted as a histogram with a bandwidth of 0.1 μm in R (ref. 60 ). The nuclear peripheral zone was defined as the area within 0.2 μm of the nuclear edge. The percentage of the padlock FISH signals localized within the nuclear peripheral zone was calculated for each independent experiment, and the means of the percentages and the s.e. are shown in the figures. The normality of the data was tested in R with a Quantile–Quantile plot, and the statistical significance between gene distribution data was tested using Welch’s two-sample t -test. RNA extraction and qRT–PCR RNA extraction and quantitative reverse transcriptase (RT)–PCR were performed as previously described [61] . Total RNA from seedlings of the indicated genotypes and growth conditions was isolated using the Spectrum Plant Total RNA Kit (Sigma, Saint Louis, MO). Complementary DNA was synthesized from messenger RNA using the Superscript II First-Strand cDNA Synthesis Kit (Invitrogen, Carlsbad, CA) according to the manufacturer’s protocol. qRT–PCR was then performed with FastStart Universal SYBR Green Master Mix (Roche, Indianapolis, IN) in a Mastercycler ep Realplex thermal cycler (Eppendorf, Hauppauge, NY). Genes and primer sets used for qRT–PCR are listed in Supplementary Table S2 . How to cite this article: Feng, C.-M. et al . Light-regulated gene repositioning in Arabidopsis . Nat. Commun. 5:3027 doi: 10.1038/ncomms4027 (2014).